Atlastin-1 regulates morphology and function of endoplasmic reticulum in dendrites Endoplasmic reticulum (ER) is characterized by interconnected tubules and sheets. Neuronal ER adopts specific morphology in axons, dendrites and soma. Here we study mechanisms underlying ER morphogenesis in a C. elegans sensory neuron PVD. In PVD soma and dendrite branch points, ER tubules connect to form networks. ER tubules fill primary dendrites but only extend to some but not all dendritic branches. We find that the Atlastin-1 ortholog, atln-1 is required for neuronal ER morphology. In atln-1 mutants with impaired GTPase activity, ER networks in soma and dendrite branch points are reduced and replaced by tubules, and ER tubules retracted from high-order dendritic branches, causing destabilized microtubule in these branches. The abnormal ER morphology likely causes defects in mitochondria fission at dendritic branch points. Mutant alleles of Atlastin-1 found in Hereditary Spastic Paraplegia (HSP) patients show similar ER phenotypes, suggesting that neuronal ER impairment contributes to HSP disease pathogenesis. The endoplasmic reticulum (ER) forms a continuous intracellular membrane system, consisting of the nuclear envelope, flat sheets, and elaborate network of tubules throughout cytoplasm [1] , [2] . ER functions in a number of essential cellular processes such as synthesis of transmembrane and secreted proteins, post-translational modification of proteins, lipid synthesis, and Ca 2+ homeostasis [3] . The highly complex and dynamic morphology of ER is important for its functions. A number of proteins have been implicated in the morphogenesis of ER [4] , [5] . The integral membrane protein Rtn4a/NogoA, a member of the ubiquitously expressed Reticulon family, functions in generating tubular ER [6] . Reticulon interacts with DP1/Yop1p, a conserved integral ER membrane protein to stabilize ER tubules by maintaining membrane curvature [6] . The ER localized dynamin-like GTPase Atlastin-1 (ATL) promotes the fusion between tubules to form ER networks [7] , [8] . ATL is highly conserved during evolution with homologs in yeast (Sey1) and plants (RHD3) [9] . Additional proteins including Climp-63, Kinectin, p180, Lunapark, and Protrudin have also been implicated in establishment and maintenance of ER morphology [10] , [11] , [12] . Differentiated cells adopt cell type specific ER morphology. For example, muscle cells use the specialized form of ER, sarcoplasmic reticulum (SR), to achieve tight coupling of membrane depolarization and contraction [13] . In yeast and plant cells, a large portion of the ER is concentrated underneath the plasma membrane [14] . In neurons, ER contains mainly tubular form in axons [15] , and both networks and tubules in dendrites [16] , [17] . ER complexity within dendrites increases at branch points in mammalian neurons [18] . The molecular mechanisms that generate and maintain the specific ER morphology in the dendrites are not fully understood. Impairment of ER function might be related to many human diseases such as Hereditary Spastic Paraplegia (HSP). HSP is a neurological disorder with progressive spasticity and weakness of the lower extremities [19] . More than 50 genetic loci have been found to be genetic causes of HSP [20] . Interestingly, many mutations in Atlastin-1 are found in HSP patients, suggesting that ER morphology might be affected in neurons of HSP patients [21] . Indeed, a series of studies have examined the function of Atlastin in axonal ER. In Drosophila motor neurons, downregulation or overexpression of Altastin cause reduced spontaneous release and the reserved pool of synaptic vesicles [22] . In another study, in Altastin mutants, ER networks in the Drosophila motor axon terminal become fragmented [23] . While the majority of the literature has focused on Altastin’s function in the axonal ER, several papers also examine its potential function in dendrites. In one study, overexpression of a GTPase dead form of Atlastin-1 in neurons leads to a decrease of ER in dendritic spines and reduced protein synthesis [24] . In another study, overexpression of wild type but not a GTPase defective form of Atlastin-1 in cortical neurons causes increased growth and branching of dendrites, suggestive of a function in dendrite morphogenesis. However, the relationship between neuronal ER impairment, Atlastin-1 and HSP has not been directly established. The PVD neuron of C. elegans is a sensory neuron with elaborate dendritic arbors. The PVD dendrite consists of stereotyped, orthogonally oriented primary, secondary, tertiary, and quaternary branches [25] , [26] . In this study, we use the PVD neuron as a model to study ER morphology and function in dendrites. Using a forward genetic screen, we isolated atln-1 mutants, which showed reduced ER tubules in the dendrite branches. We found that atln-1 mutant had impaired GTPase activity and was unable to fuse membrane both in vivo and in vitro. We also report that the abnormal ER morphology led to defects in mitochondria attachment and fission at dendritic branch points and abnormalities in protein homeostasis when the unfolded protein response (UPR) was compromised. Mutant alleles of Atlastin-1 found in HSP patients showed similar ER defects, suggesting that neuronal ER impairment contributes to HSP pathogenesis. ATLN-1 is required for ER tubule extension into dendrites To visualize the ER morphology in the PVD neuron, we expressed the ER residential protein: signal peptidase (SP12) [27] fused with GFP with a PVD specific promoter, ser-2 Prom3 [28] , [29] , [30] . Using Three-Dimensional Structured Illumination Microscopy (3D-SIM), we observed that the GFP fluorescence pattern in the PVD soma exhibited a typical ER pattern, including a nuclear envelope and sparse connected tubule networks (Fig. 1a ). Consistent with previous reports, ER extended to both axon and dendrites (Fig. 1b, c ). Surprisingly, within dendrites, ER was only found in a subset of dendritic branches. ER filled the entire length of the primary dendrites, but only extended to a fraction of the secondary (2°) and tertiary (3°) dendrites, and very rarely extended to tertiary (4°) dendrites (Fig. 1b, c ). The number of 2° branches containing ER gradually increased after the entire dendritic branches formed at L4 stage, indicating that the ER extension to the dendritic branches significantly trailed dendrites formation (Fig. 1i ). To validate the SP12 marker, we also expressed several other ER proteins such as ESYT-2 and SEC-61 fused with GFP in PVD. They both showed similar patterns as GFP::SP12 in both the PVD soma and dendrites (Supplementary Fig. 1E, G and J ). Fig. 1 ATLN-1 is required for ER invasion into dendrites. a A representative 3D-SIM image of ER (GFP::SP12) in wild-type PVD soma (A single focal plane is shown). The yellow arrow indicates the nuclear membrane and the white arrow indicates a tubular network. Scale bar, 1 μm. b A schematic picture showing that ER extends into some but not all 2° and 3°dendrites in PVD. Magenta lines represent PVD dendritic branches and green lines indicate ER distribution. c , d Representative confocal images of ER (GFP::SP12) and dendritic morphology of PVD neuron ( ser-2 P3::mCherry) in wild type ( c ) and atln-1 ( wy50080 ) mutant ( d ) at L4 stage. Arrows show PVD 2° branches without ER and arrowheads indicate PVD 2° branches with ER. Asterisks mark the PVD axon. Scale bars, 10 μm. e–h Representative ER morphology of PVD neuron in WT ( e ), atln-1 ( f ) , atln-1; ser-2 Prom3:: atln-1 #2 (transgenic line #2) ( g ) and atln-1; ser-2 Prom3:: atln-1 K80A #1(transgenic line #1) ( h ) at adult stage. Scale bars, 10 μm. i , j Quantification of ER 2° branches number. Values are mean and error bars are SEM, n = 46 for each genotype. * p < 0.05; *** p < 0.001 (two-sided student’s t test and Tukey’s multiple comparison test) Full size image To understand the molecular mechanisms underlying ER distribution in dendrites, we carried out an unbiased, forward genetic screen using this ER marker. From about 4000 mutated haploid genomes, we isolated 12 mutants with abnormal ER pattern. Among them, the wy50080 mutant showed dramatically reduced ER tubules in 2° and 3° dendrites at all developmental stages compared to the wild type, regardless of the ER markers (Fig. 1c–f, i ; Supplementary Fig. 1E–I ). Using SNP mapping and sequencing, we identified the causative mutation in the atln-1 gene, the ortholog of the vertebrate Atlastin-1 (Supplementary Fig. 1A ). PVD specific expression of atln-1 rescued the ER phenotype of wy50080 (Fig. 1g, j ), indicating that atln-1 functioned cell-autonomously in PVD to regulate ER morphology. In non-neuronal cells, Atlastin-1 is an ER localized GTPase that establishes ER networks by mediating homotypic membrane fusion [7] , [8] . To test if the GTPase activity of ATLN-1 was essential for its function in ER morphology in PVD, we introduced the K80A mutation into altn-1 , a mutation that disrupts GTP binding in the vertebrate Atlastin-1 [31] . The ATLN-1 K80A transgene failed to fully rescue the ER phenotype in the atln-1 mutants (Fig. 1h, j ), indicating that the GTPase activity of ATLN-1 is critical for dendritic ER morphology. The subtle rescue activity might be due to the partial allelic complementation between the two mutant alleles. The mutation in atln-1(wy50080 ) is a missense mutation that causes the amino acid substitution P219L, which localizes in the GTPase domain. We used in vitro assays to test whether this mutation affected the GTPase activity as well as the membrane tethering and fusion activity. We introduced the corresponding mutation P183L in the Drosophila ortholog dmATL and used a previously characterized K51A mutation as a positive control. The K51A mutation was shown to reduce GTPase activity and completely lack tethering and fusion activity [8] , [32] . Interestingly, the GTPase activity of P183L mutant was drastically reduced, similar to that of K51A (Fig. 2a ). Wild-type and mutant dmATL were then purified and reconstituted into vesicles for membrane tethering and fusion activity analyses (Fig. 2b ). Tethered vesicles caused an increase in turbidity, which could be monitored by measuring light absorbance at 405 nm (Fig. 2c ). A fluorescence de-quenching assay was used to determine fusion activity based on lipid mixing. The donor vesicles contained lipids labeled with both nitrobenzoxadiazole (NBD) and rhodamine at quenching concentrations. Once fused with acceptor vesicles, the labeled lipids became diluted, resulting in increase in NBD fluorescence (Fig. 2d ). Similar to K51A, P183L mutant completely lacked membrane tethering and fusion activity (Fig. 2c, d ). Thus, P183L behaved indistinguishably as K51A in all three assays, indicating that the atln-1 mutant (P219L) should have dramatically reduced GTPase activity and might have defects in ER tubule fusion and networks formation. Fig. 2 ATLN-1 regulates somatic ER network formation. a Quantification of GTPase activity of WT and mutant dmATLs. The activities were measured by phosphate release at saturating GTP concentrations of 0.5 mM. At least three repetitions were performed for each group. Values are mean and error bars are SEM. ns, not significant; *** p < 0.001 (Tukey’s multiple comparison test). b Reconstitution of Drosophila WT, P183L, and K51A dmATL proteins into liposomes. Donor ( D ) and acceptor ( A ) vesicles with recombinant proteins were analyzed by SDS/PAGE and Coomassie blue staining. ( c ) Schematic illustration of liposome membrane tethering assay (upper panel). The clustering of Drosophila WT and mutant dmATL containing proteoliposomes (protein:lipid ratio 1:2,000) was measured by the light absorbance at a wavelength of 405 nm (lower panel). d Schematic illustration of lipid mixing assay (upper panel). Drosophila WT and mutation dmATL were reconstituted at equal concentrations into donor and acceptor vesicles. GTP-dependent fusion of donor and acceptor vesicles was monitored by the dequenching of an NBD-labeled lipid in the donor vesicles (lower panel). Fusion was initiated by addition of GTP. e Representative 3D-SIM image of PVD somatic ER in a WT worm (single focal plane). f – h Representative 3D-SIM maximum-intensity-projection images of PVD somatic ER in WT ( f ), atln-1 ( g ) and atln-1; ser-2 P3:: atln-1 worms at adult stage. Insets show 2X magnified views. The magenta arrows indicate three-way junction and white arrows indicate parallel ER tubules. Scale bar, 1 μm Full size image Atlastin-1 functions as dimer when mediating homotypic ER membrane fusion [7] . Most Atlastin-1 mutations found in HSP patients are heterozygous mutations that function as dominant negative alleles to further inhibit the function of the wild-type allele. To distinguish whether the P219L allele was a loss-of-function or dominant negative allele, we overexpressed the mutant P208L (P208L is the equivalent mutation in the mammalian ATL1) as well as the known K80A ATL1 in wild-type COS-7 cells, which endogenously express the ATL2 and ATL3 paralogs but not ATL1 itself. As expected, the K80A ATL1 caused a reduction in the density of 3-way junctions of the ER networks due to its dominant negative effects. The P208L ATL1 did not show a similar detrimental effect (Supplementary Fig. 2A ). We further tested if P208L was a loss-of-function mutant with rescue experiments. COS-7 cell lines lacking both ATL2 and ATL3 showed reduced density of ER 3-way junctions. This phenotype could be rescued by wild-type ATL1 but not the P208L or K80A forms, further confirming that the P208L allele represented a loss-of-function allele (Supplementary Fig. 2B ). To test if the worm P219L atln-1 behaved similarly in PVD, we expressed the atln-1 (P219L) in wild-type PVD and observed no dominant negative effect (Supplementary Fig. 2F–H ). Furthermore, we did not observe any ER phenotype in the atln-1 mutant (P219L) heterozygotes (Supplementary Fig. 2E, H ). Together, these data indicate that P219L is a loss-of-function allele. To directly test if ATLN-1 was required for ER membrane fusion in neurons, we imaged the ER networks in the PVD soma using 3D-SIM. In wild-type controls, ER formed complex networks characterized by numerous three-way junctions (Fig. 2e, f ). While in atln-1 mutants, the ER networks were visibly less complex with fewer three-way junctions and dramatically increased parallel, unbranched ER tubules (Fig. 2g ). This ER morphology defect was rescued by a wild-type ATLN-1 transgene expressed in PVD (Fig. 2h ). Both the reduction of ER networks and the appearance of parallel tubules in the altn-1 mutant were strikingly similar to the ER defects in mammalian non-neuronal cells lacking Atlastin-1 [7] . Consistent with its ER shaping function, we found that GFP::ATLN-1 was localized to numerous tubule structures in the cell body and tubules in the dendrites that highly resembled the ER pattern in the PVD soma and dendrites (Supplementary Fig. 1B–D ). Together, these evidences suggest that ATLN-1 is localized on neuronal ER and is required to establish somatic ER tubule networks in PVD. atln-1 mutant causes excessive ER retraction in PVD To understand why ER branches were reduced in PVD dendrites in the atln-1 mutants, we performed time-lapse imaging experiments to record the ER (GFP::SP12) dynamic in PVD tertiary dendrites. In wild-type worms, some ER tubules showed a dynamic pattern characterized by growth and retraction, while others were stable during the imaging experiments (Fig. 3a ). In atln-1 mutants, we found that the frequency of ER extension into the branches was not changed, but the retraction frequency was increased when compared with wild-type worms (Fig. 3a, b, d ). PVD specific expression of ATLN-1 could fully rescue this phenotype (Fig. 3c, d ). Also, we found that both the growth and retraction length were increased, which was fully rescued by PVD specific expression of atln-1 (Fig. 3e, f ). These results suggest that the reduction of ER in dendritic branches in atln-1 mutants might be caused by excessive retraction. Fig. 3 a tln-1 mutants show high level of ER retraction. a – c Kymographs of ER (GFP::SP12) dynamic events in PVD 3° branches in WT ( a ), atln-1 ( b ), and atln-1; ser-2 P3:: atln-1 ( c ) worms at L4 stage. Magenta, white and yellow arrows indicate ER growth, retraction, and static events, respectively. Scale bar, 5 μm and 10 s. d Quantification of ER growth and retraction frequency. Values are mean and error bars are SEM. At least 200 events from more than 30 worms are quantified. ns, not significant, ** p < 0.01 (Newman-Keuls multiple comparison test). e, f Quantification of ER growth ( e ) and retraction ( f ) length. Values are mean and error bars are SEM. At least 200 events from more than 30 worms are quantified. ns, not significant; *** p < 0.001 (Newman-Keuls multiple comparison test). g – i Representative 3D-SIM images of ER (GFP::SP12) complex structure at the most proximal branch point of the PVD anterior dendrite in WT ( g ), atln-1 ( h ), and atln-1; ser-2 P3:: atln-1 ( i ) worms. j Quantification of ER complexity index of the most proximal branching point. Values are mean and error bars are SEM, n > 40. ** p < 0.01; *** p < 0.001 (Newman-Keuls multiple comparison test). To calculate the complexity index, we drew a circle of 1.6 μm diameter (dashed circle) at the branching point and a line within the circle along the dendrite trunk (dashed line). Complexity index = mean GFP intensity in the circle/mean GFP intensity on the line. Scale bars, 1 μm. k Quantification of ER complexity index at posterior branch points. Values are mean and error bars are SEM. At least 100 branch points from more than 30 worms are quantified. * p < 0.05; *** p < 0.001 (Newman-Keuls multiple comparison test). l Scanning electron microscopy images from a serial EM pictures showing ER complex structure on a branch point in PVD of a WT worm. The magenta arrows indicate ER. The blue arrows indicate PVD 2° branches. Scale bar, 500 nm Full size image Next, we investigated why ER tubules retracted from dendrite branches in atln-1 mutants. The ER tubules in branches originated from tubules in the primary dendrite. We noticed that ER formed small network structures at the branch sites where the volume of the neurites were greater compared with the dendritic trunk (Fig. 3g ). Using “automatic collector of ultrathin sections scanning electron microscopy” (AutoCUTS-SEM) [33] , we reconstructed a segment of the PVD primary dendrite containing a 2° branch site. The ultrastructure showed that there were multiple ER cross section-like profiles at the branch site, consistent with a small ER network (Fig. 3l ). Using the super-resolution SIM imaging, we found that the ER networks at the branch points were replaced by unbranched tubules in atln-1 mutants, which was rescued by PVD expression of atln-1 (Fig. 3h–k ), indicating a key role of atln-1 in formation of ER networks at branch points. Since ER tubules in 2° dendrites originated from the ER networks at branch points, we speculated that ER networks might promote ER tubules formation or stabilization in 2° dendrites. To test this hypothesis, we divided branch points (BPs) into two types: the ones with ER tubules extending into the corresponding 2° dendrites (+ER BPs) and the ones without ER tubules in the 2° dendrites (−ER BPs). We then compared the ER complexity at these two types of BPs. More complex ER networks were found in the +ER BPs compared to the −ER BPs (Supplementary Fig. 3A–C ), which is consistent with the notion that ER networks at BPs may help to stabilize ER tubules in the 2° dendrites. ER and microtubules (MTs) mutually affect each other in dendrites In non-neuronal cells, ER tubules extend along MTs using sliding mechanism or tip attachment complex (TAC) mechanism [34] . To investigate if the ER extension defect in atln-1 mutants was related with MTs, we expressed the α-tubulin protein TBA-1 fused with GFP to monitor MT’s pattern and dynamics in PVD [35] . Interestingly, MTs showed very similar pattern as ER in PVD dendrites: both ER and MTs were present in a fraction of secondary and tertiary dendrites (Supplementary Fig. 4B ). Our unpublished results showed that ER extension into the PVD 2° and 3° branches was strictly dependent on the transient presence of MTs during the ER outgrowth events, while retraction of ER from the branches was not (unpublished results X. L., X. W. and K. S.). Further, co-localization analyses showed that ER and MTs were mostly present in the same branches, and atln-1 mutants did not change the co-localization of ER and MTs (Supplementary Fig. 4A–D ), consistent with the notion that ER might enter the branches through a MTs dependent mechanism. We also noticed that MTs (GFP::TBA-1) within the 2° and 3° branches were significantly reduced in the atln-1 mutants compared with wild-type controls (Fig. 4a, b, d ). This phenotype was found in both L4 and adult worms and could be largely rescued by PVD expression of wild-type atln-1 , suggesting that ATLN-1 affects MTs distribution in dendritic branches (Fig. 4c, d ). Fig. 4 ATLN-1 affects the presence of MT in dendritic branches. a – c Representative confocal images of MTs (GFP::TBA-1) and dendritic morphology of PVD neuron ( ser-2 P3::mCherry) in WT ( a ), atln-1 ( b ), and atln-1; ser-2 Prom3:: atln-1 adult worms ( c ). Arrows show PVD 2° branches without MTs and arrowheads indicate PVD 2° branches with MTs. Scale bars, 10 μm. d Quantification of the number of 2° branches with MTs. Values are mean and error bars are SEM, n > 40. ns, not significant; *** p < 0.001 (Newman-Keuls multiple comparison test) Full size image To further understand ATLN-1’s role in MT regulation, we conducted time-lapse imaging experiments to study the MTs’ dynamic behavior in tertiary branches. MTs were sparsely distributed in 3° branches, providing us with the resolution to visualize single MT filament [36] , [37] . From kymograph analyses, we could often observe the distinct dynamic behaviors of two ends of the same MTs (TBA-1::GFP, Fig. 5a ). We designated the more dynamic ends as the plus-ends and the more stable ends as minus-ends (Fig. 5a ). To understand the relationship between ER and MTs, we further divided MTs into two categories: MTs that overlap with an ER tubule (+ER) or do not overlap with ER (−ER) in the 3° branches (Fig. 5a ). Fig. 5 MT dynamics and numbers are affected by the ER. a Kymographs recording the dynamic events of MT (GFP::TBA-1) and ER (mCherry::SP12) in 3° branches from a L4 stage WT animal. A blue box labels a +ER MT, while an orange box labels a –ER MT. MT’s plus end is marked by (+) and minus end is marked by (−). Scale bar, 5 μm and 15 s. b – e Quantification of dynamic parameters of MT plus ends ( b , d ) and minus ends ( c , e ). The frequency of rescue ( b , c ) and catastrophe ( d , e ) were plotted. Values are mean and error bars are SEM. At least 150 events from more than 30 worms are quantified. ns, not significant; * p < 0.05; ** p < 0.01; *** p < 0.001 (Newman-Keuls multiple comparison test). f Confocal images showing tdTomato::PTRN-1 puncta in PVD 3° branches at adult stage. +ER (in blue box) means a 3° dendrite with ER present. -ER (in orange box) means the 3° branch without ER present. Scale bars, 10 μm. g Quantification of PTRN-1 puncta density in −ER and +ER 3° dendrites. Values are mean and error bars are SEM. At least 100 confocal views of PVD proximal regions from more than 40 worms are quantified. *** p < 0.001 (two-sided student’s t test) Full size image In wild-type animals, we found that the growing ends of MTs were less dynamic for +ER MTs compared with the −ER MTs. This was reflected by decreased frequency of both MTs catastrophe and rescue in the +ER MTs (Fig. 5a–e ). C. elegans neurites contain partially tiled MT arrays. The number of MTs can be estimated by the density of minus-end marking PTRN-1 puncta along the neurites [37] , [38] . We found that the density of PTRN-1 puncta was higher in the +ER 3° branches compared to that of the –ER 3° branches (Fig. 5f, g ). The +ER and –ER branches are indistinguishable from each other in morphology, and are both dependent on the same molecular pathways for their development [29] , [39] . These observations suggest that ER might stabilize nearby MTs in dendritic branches. Since Atlastin has been shown to recruit MT severing enzyme spastin [40] , we next asked if MT dynamics were changed in the atln-1 mutants. For the –ER MTs, we did not detect any difference between WT and atln-1 mutants, strongly suggesting that atln-1 does not directly regulate MT dynamics in PVD. For the +ER MTs, we found that altn-1 mutant MTs’ plus-ends were slightly more stable compared to WT, suggesting that ATLN-1’s effect on MTs might be through affecting ER structure and function. These phenotypes were fully rescued by expression of wild-type ATLN-1 in PVD (Fig. 5b, d ). Together, these results suggest that ER could stabilize adjacent MTs. ATLN-1 modulates mitochondria behavior in dendrites Above evidences showed that ALTN-1 was required for ER morphogenesis in the neuronal cell body and dendrites. Since ER is an expansive network and has been shown to contact other organelles and perform many cellular functions, we investigated if the ER morphology affected its functions. Interaction between ER and mitochondrion could enhance mitochondrion fission [41] . In neurons, ER-mitochondria contacts are critical for Ca 2+ regulation [42] . To assess if the impairment of ER in atln-1 mutant would affect mitochondria pattern in PVD dendrites, we marked mitochondria by expressing TOMM-20 (1-54aa)::GFP in PVD. We found that mitochondria were highly enriched at the dendritic branching sites: more than 50% of mitochondria in the primary dendrite were localized to the PVD dendritic branch sites at different developmental stages in wild-type worms (Fig. 6a, d ). Since the branch sites contained ER networks, we hypothesized that mitochondria might be enriched there due to the local ER network. Fig. 6 ATLN-1 modulates mitochondria dynamics in dendrites. a – c Mitochondria distribution in PVD primary dendrites in WT ( a ), atln-1 ( b ) and atln-1; ser-2 Prom3:: atln-1 ( c ) worms at adult stage. Arrows indicate mitochondria at branch points. Arrowheads indicate mitochondria which are not localized at branch points. Scale bar, 5 μm. d Quantification of the percentage of mitochondria localized at branch points. Values are mean and error bars are SEM, n > 25 for each genotype. ns, not significant; * p < 0.05; ** p < 0.01; *** p < 0.001 (Newman-Keuls multiple comparison test). e – g Time-lapse images of mitochondria fission in WT ( e ), atln-1 ( f ), and atln-1; ser-2 P3:: atln-1 ( g ) worms. The arrows indicate mitochondria fission events at branch points. The arrowheads indicate mitochondria fission events outside of branch points. Scale bar, 10 μm. h Quantification of mitochondria fission events at and outside of branch points. n = 40–50. ns, not significant; * p < 0.05 (Chi-square test) Full size image To test this idea, we examined the mitochondria localization in the atln-1 mutants where the branch sites localized ER networks were less complex. Compared with wild-type worms, the number of mitochondria localized to branch points was decreased at all the developmental stages in atln-1 mutants (Fig. 6b, d ). Since most mitochondria fission events occurred at ER-mitochondria contact sites [43] , we wondered if mitochondria fission might preferentially occurred at the branching sites and might be dependent on atln-1 . Consistent with this hypothesis, mitochondria fission events at PVD dendritic branch sites were reduced from 66 to 41% in atln-1 mutants (Fig. 6e, f, h ). These phenotypes could be rescued by expression of wild-type ATLN-1 (Fig. 6c, d, g, h ). In summary, these data suggest that local ER network at dendrite branch sites might anchor mitochondria and promote mitochondria fission. atln-1 functions synergistically with ire-1 The inositol-requiring enzyme 1 (IRE1) senses the ER stress and activates the UPR pathway [44] . Perturbation of the IRE1 arm of the UPR pathway causes loss of PVD dendritic branches [45] . We speculated that ER loss in PVD dendrites of atln-1 mutant might further impair the ER function and block UPR. To test this idea, we constructed double mutants between ire-1 and atln-1 . Interestingly, the double mutants showed enhanced PVD dendrite arborization defect, although atln-1 mutant alone did not show any visible dendrite morphogenesis phenotype (Fig. 7a–e ). Fig. 7 a tln-1 functions synergistically with ire-1 . a – d Representative confocal images of PVD ( ser-2 P3::GFP) morphology in WT ( a ), atln-1 ( b ), ire-1 ( ok799 ) ( c ) and atln-1; ire-1 ( d ) worms at adult stage. Scale bars, 10 μm. e Quantification of the number of PVD 2° branches. Values are mean and error bars are SEM, n > 40. ns, not significant; *** p < 0.001 (Newman-Keuls multiple comparison test). f – i Confocal images of DMA-1::GFP in PVD cell body in WT ( f ), atln-1 ( g ), ire-1 ( h ), and atln-1; ire-1 ( i ) worms. Arrows indicate DMA-1::GFP puncta. Scale bar, 5 μm. j Quantification of DMA-1::GFP fluorescence intensity in PVD cell body. Values are mean and error bars are SEM, n = 40–50. ns, not significant; *** p < 0.001 (Newman-Keuls multiple comparison test). k – n Confocal images of DMA-1::GFP in anterior primary dendrite around the PVD soma in WT ( k ), atln-1 ( l ), ire-1 ( m ), and atln-1; ire-1 ( n ) worms. Arrows indicate DMA-1::GFP puncta. Asterisk marks cell body. Scale bar, 5 μm. o Quantification of DMA-1::GFP fluorescence intensity of primary dendrites in ( k – n ). Values are mean and error bars are SEM, n = 40–50. ns, not significant; *** p < 0.001 (Tukey’s multiple comparison test) Full size image We have previously shown that the UPR pathway is required to fold and deliver the dendrite arborization receptor DMA-1 [45] . In wild-type animals, DMA-1::GFP was largely localized to secretory vesicle-like structures in the soma and showed  a diffuse plasma membrane-like pattern in the dendrites (Fig. 7f, k ). In ire-1 mutants, DMA-1 was largely trapped in the ER and reduced on the dendritic plasma membrane, especially at distal dendrites (Fig. 7f–h, j and Wei et al., 2015), leading to failed distal dendrites formation. Interestingly, in ire-1 ; atln-1 double mutants, the overall level of DMA-1::GFP was greatly reduced compared with the ire-1 single mutants (Fig. 7h–j ). The dim DMA-1 signal still exhibited a predominant ER staining pattern in PVD soma (Fig. 7i ). In the double mutants, even the proximal dendrites were nearly completely devoid of DMA-1 signal (Fig. 7k–o ), which likely caused the enhanced dendrite arborization defect. These results suggest that ER networks morphology might affect homeostasis of neuronal membrane proteins and this requirement is particularly important when UPR is compromised. HSP disease alleles of Atlastin-1 affect ER morphology Hereditary Spastic Paraplagia (HSP) is a class of diseases characterized by the neuronal degeneration of peripheral nervous system. A number of missense mutations of Atlastin-1 have been reported in HSP patients [46] . The pathogenic mechanisms of these mutations are not fully understood. Interestingly, other HSP genes such as Reticulon and REEP affect ER morphology in Drosophila axons [47] . Next we asked if HSP disease mutations of Atlastin-1 affected dendritic ER pattern in PVD. We chose three Atlastin-1 mutations found in HSP patients, F151S, I315S, and S519N, which localized to different domains of Atlastin-1. The corresponding conserved mutation sites in C. elegans were F161S, I326S, and S530N, respectively (Fig. 8a ). We overexpressed these three disease alleles, the wild-type atln-1 , and the GTPase defective K80A allele in wild-type worm’s PVD and examined the ER morphology in each genotype. As a control, overexpression of the wild-type atln-1 did not show any ER phenotype (Fig. 8b, g ). However, overexpression of all three HSP alleles and K80A caused reduced ER in the secondary and tertiary branches similar to the phenotypes found in the loss-of-function atln-1(wy50080) mutants (Fig. 8c–g ). In addition, expression of F161S and I326S also caused striking ER morphology phenotypes in the PVD soma characterized by a reduction of ER networks and increased parallel ER tubules (Fig. 8h–j ). Together with the human genetics literatures, these results support the notion that neuronal ER morphology defects contribute to the pathogenesis of HSP. Fig. 8 HSP disease alleles of Atlastin-1 affect ER morphology. a Schematic diagram of ATLN-1 protein domains. K80A, wy50080 (P219L) and HSP related disease mutations are showed. b – f Representative ER morphology in Ex[ ser-2 P3:: atln-1 ] ( b ), Ex[ ser-2 P3:: atln-1 K80A ] ( c ), Ex[ ser-2 P3:: atln-1 F161S ] ( d ), Ex[ ser-2 P3:: atln-1 I326S ] ( e ) and Ex[ ser-2 P3:: atln-1 S530N ] ( f ) transgenic adult worms. Scale bars, 10 μm. g Quantification of ER 2° branches number. Values are mean and error bars are SEM, n = 40–50. ns, not significant; ** p < 0.01; *** p < 0.001 (Tukey’s multiple comparison test). h , i Representative maximum-intensity-projection 3D-SIM images of ER in PVD soma in Ex[ ser-2 P3:: atln-1 F161S ] ( g ) and Ex [ ser-2 P3:: atln-1 I326S ] ( h ) transgenic adult worms. Insets show 2X magnified views. Scale bar, 1 μm. j Quantification of 3-way junctions in a 3 μm 2 region at anterior primary dendrite initiation segment (the dashed boxes in h and i ). Values are mean and error bars are SEM, n > 30. ns, not significant; *** p <0.001 (Newman-Keuls multiple comparison test) Full size image ER shaping and HSP genes are required in ER invasion There are three Atlastin proteins ATL1, ATL2, and ATL3 in mammals, which function redundantly to modulate ER morphology [48] . C. elegans genome encodes two Atlastin homologs atln-1 and atln-2 . In PVD, atln-2 was not required for ER morphology as atln-2(wy50125) mutant did not show any ER phenotype (Supplementary Fig. 5A and C ) and atln-1(wy50080) ; atln-2(wy50125) double mutants did not enhance atln-1(wy50080) single mutant’s phenotype (Supplementary Fig. 5B and C ). These results suggested that atln-1 but not atln-2 was essential in regulating ER morphology in PVD. To address whether atln-2 is expressed in PVD, we constructed two 2 kb promoters driven GFP ( atln-2 Prom1::GFP and atln-2 Prom2::GFP) to monitor the expression pattern of different atln-2 isoforms. Both of the constructs showed expression in a single head neuron but not in PVD (Supplementary Fig. 5D–G ). Therefore, the lack of expression in PVD might explain why PVD ER morphology is normal in the atln-2 mutants. Aside from ATLs, ER tubules are shaped by the curvature-stabilizing proteins such as Reticulons and REEPs, which are HSP associated proteins [5] . These ER shaping proteins are known to have similar activity and redundant functions [5] . We systematically examined the ER phenotype in mutant alleles for these genes including yop-1(tm3667) (REEP5 and REEP6 ortholog), ret-1(tm390) (reticulon ortholog), and T19C3.4(wy50209) (REEP1-4 ortholog) in PVD. Each mutant showed subtle ER extension defects (Supplementary Fig. 6A, C, D and K ). In addition, lnp-1(wy50227) , the mutant of another ER shaping protein Lunapark, which functions to stabilize nascent three-way junctions [49] , also showed decreased ER of PVD dendrites (Supplementary Fig. 6E and K ). Furthermore, spas-1(tm683) , the mutant of another HSP causative gene Spastin [50] also showed ER morphology defect (Supplementary Fig. 6B and K ), although not as severe as the atln-1 ( wy50080 ) mutant. To explore the relationship between atln-1 and these genes, we constructed the double mutants between atln-1 and these genes. Only ret-1(tm390) ; atln-1(wy50080) double mutants enhanced the ER defects of atln-1 single mutants (Supplementary Fig. 6F–J and L ), suggesting ret-1 and atln-1 indeed play partially redundant functions to regulate ER extension in PVD dendrites. yop-1 , lnp-1 , spas-1 , and T19C3.4 did not enhance the phenotype of atln-1 , which might be due to additional redundant functions of other ER shaping proteins. Together, it suggests that multiple ER shaping and HSP related protein cooperate to regulate ER morphology in neurons. In this study, we use the C. elegans sensory neuron PVD to understand how cell type specific ER morphology is established in dendrites and whether the specific morphology is related to its function in neurons. Our current study adds to the understanding of Atl1 in the following aspects. First; we systemically examine the ER morphology and dynamics in dendrites in vivo. Second; our results suggest that ER and MTs mutually influence each other in dendrites: while MT dynamics and motor proteins mobilize ER extension into dendritic branches, ER also functions to stabilize MTs. Third; we show that complex ER networks at dendritic branch points modulate mitochondria fission and localization. Fourth, we show that ATLN-1 regulates protein homeostasis when UPR is impaired. Fifth, we have examined the impact of many HSP mutant alleles in dendritic ER morphology in our system and show that ER impairment in neurites might be the cause of HSP. In the PVD soma, ER forms network pattern, similar to non-neuronal cells, while PVD dendrites mainly contain ER tubules. This type of distribution pattern is similar to what has been observed in the mammalian neuron’s cell body and axon [2] , [15] . Interestingly, we notice that the ER complexity increase with the appearance of small ER networks at dendrite branch points. It is shown that more complex ER networks form at the branch sites of dendrites in culture mammalian neuronal cells [18] . These similarities argue strongly that the ER networks at dendrite branching points are conserved features of dendrites and are likely to have functional significance. In order to understand the structure function relationship between the morphology and function of ER, we search for molecular manipulations that can change critical aspects of ER morphology in neurons. Interestingly, the unbiased genetic approach leads us to the usual suspect of ATLN-1. atln-1 mutants reduce the complexity of ER likely by preventing tubules fusion and three-way junctions formation. In atln-1 mutants, ER has less branched network structures and more parallel tubules. This change is apparent at both cell body and the dendritic branch points. Next, we ask if these ER morphology changes lead to functional deficits in atln-1 mutants. First, related to the reduction of ER networks at dendrite branch points, we find reduced ER tubules in the corresponding dendritic branches. Interestingly, in atln-1 mutants, ER tubules’ growth into dendritic branches is not affected. Instead, the retraction of tubules from dendrite branches is increased compared with wild-type animals. These results suggest that the ER networks might be required for stabilizing the ER tubules that extend into the 2° dendrites. It is conceivable that the ER networks at the branch sites modulate the ER membrane tension, which affects the stability of ER tubules. Second, we find that mitochondria are enriched at the dendrite branch points. More than half of the mitochondria are localized nearly to branch points, which is dramatically different from a random pattern. This branch point enrichment is reduced in atln-1 mutants, suggesting that the ER networks might contribute to anchoring of mitochondria either through physical hindrance of trafficking or specific molecular interactions between mitochondria and ER. In wild-type animals, we also observe that mitochondria undergo fission preferentially at the branch points. Since ER-mitochondria contact has been shown to facilitate mitochondria fission [41] , it is likely that the ER networks at the branch points provide a platform for mitochondria anchoring and fission. Together with the previous evidences showing the complex ER structure at branch points enriches protein synthesis and secretion machinery [18] , our data broadens the potential function of branch point ER networks. Third, related to the somatic ER networks, we find that the level of the dendrite receptor protein DMA-1 is significantly reduced in the atln-1 mutant under ER stress conditions. Consequently, the dendrite branching phenotype of ire-1 mutant is significantly enhanced by the atln-1 mutation. Since the vast majority of ribosomes are found in the soma (Supplementary Fig. 7 ), we postulate this defect of atln-1 mutants is due to the ER networks defect in the soma. Together, these evidences suggest that the ER networks morphology in the neuronal soma and at dendrite branch points are important for several aspects of neuronal cell biology. In wild-type animals, ER tubules extend from the branch-site networks into the 2° branches using MTs dependent mechanisms. The extension of the ER requires the presence of MTs within the branches and is likely dependent on MT motor proteins [34] . The distribution of ER tubules in dendritic branches highly correlates with the MTs distribution, suggesting that the growth of ER and MTs are related. In fibroblasts, the interaction between ER and MTs is an important determinant of ER morphology [54] . When ER is bound to MTs in fibroblasts, CLIMP63 promotes extension of ER tubules to the cell periphery along MT tracks [51] , [52] . However, we find that both ER and MTs extension into the branches are defective in atln-1 mutant. And our data show that ATLN-1 likely directly affects ER morphology and indirectly affects MT dynamics. For the ER extension defect of atln-1 mutant, Our results show that this phenotype correlates with the reduced complexity of ER networks at the branching points (Supplementary Fig. 3 ), which may directly depend on the function of ATLN-1. For the MT extension defect in atln-1 mutants, we speculate it’s a secondary effect of defective ER since we find that ER and MTs could mutually affect each other in our system. MTs are required for the entry of ER into the PVD dendritic branches. This is consistent with many previous studies in the field. Our unpublished data also show that: (1) ER entry into the 2° and 3° branches is strictly dependent on the presence of MTs in the same branches. (2) ER could enter the PVD 2° dendrites along static MTs, likely driven by MTs based motors. (3) ER could also enter together with the growing tip of MTs. Both motor mediated and tip attachment mechanisms are consistent with the mechanisms of ER movement in non-neuronal cells. (4) ER could also retract from branches, which could happen in the absence of MTs. Therefore, ER needs MTs to grow but ER retraction is not dependent on MTs. Since some branches contain MTs and others do not, the PVD dendrites provide us with an experimental system to ask whether ER can also affect the dynamic behavior of MTs. In wild-type animals, when we compare MTs in the branches with or without ER, we find that MTs grow less and shrink less in ER positive branches, indicating that the presence of ER makes MTs more stable (less dynamic) (Fig. 5a–e ). To further corroborate these results, we examine the PTRN-1 puncta as a proxy to MT numbers in –ER and +ER branches. We find that there are more PTRN-1 puncta in the +ER branches, indicating that there are more MTs in the +ER branches (Fig. 5f, g ). The fact that atln-1 mutants do not change the dynamic behavior of MTs in –ER branches suggests an indirect role of ATLN-1 on MT dynamic regulation. Additionally, atln-1 mutants show slightly more stable MT plus-ends in the +ER branches compared to the wild-type control. This effect is subtle but is statistically significant and could be rescued by cell autonomous expression of wild-type ATLN-1. Consistent with our data, Atlastin-1 has been shown to physically interact with the N terminal of MT-severing protein Spastin in Drosophila muscle, which negatively regulates MT stability [53] . Taken together, these data indicate that ER might be able to stabilize MTs in the dendrites with an unknown mechanism. Atlastin-1/SPG3A is a well-known factor in HSP, which is supported by the discoveries of many Atlastin-1 mutations in HSP patients. Introducing several mutant alleles to worms show very similar phenotype in PVD soma and dendrites as atln-1 loss-of-function mutants, suggesting the conserved function of Atlastin-1 in controlling dendrite and neuronal somatic ER morphology might contribute to HSP pathogenesis. Furthermore, mutants of several other HSP genes including YOP-1 (REEP), RET-1(reticulon) also show ER morphology defects in dendrite, indicating that neuronal ER morphogenesis defect might be a common pathological feature of HSP. Strains and genetics The wild-type strain N2 Bristol and all the mutants were cultured on the nematode growth medium (NGM) plates seeded with Escherichia coli OP50 at 20 °C following the standard protocol (Brenner, 1974). Standard cloning procedure of Clontech In-Fusion PCR Cloning System was used to construct all the plasmids. PCR products were produced by Phusion DNA polymerase (New England Biolabs) or TransStart FastPfu DNA Polymerase (Transgen Biotech) or High-Fidelity Master Mix (TsingKe Biotech) following standard procedures. 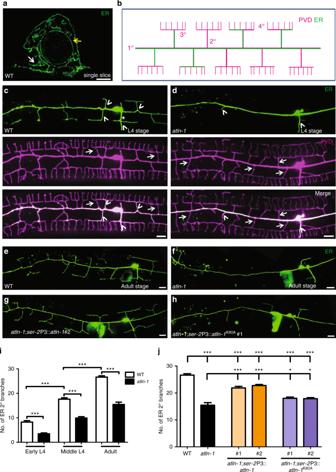Fig. 1 ATLN-1 is required for ER invasion into dendrites.aA representative 3D-SIM image of ER (GFP::SP12) in wild-type PVD soma (A single focal plane is shown). The yellow arrow indicates the nuclear membrane and the white arrow indicates a tubular network. Scale bar, 1 μm.bA schematic picture showing that ER extends into some but not all 2° and 3°dendrites in PVD. Magenta lines represent PVD dendritic branches and green lines indicate ER distribution.c,dRepresentative confocal images of ER (GFP::SP12) and dendritic morphology of PVD neuron (ser-2P3::mCherry) in wild type (c) andatln-1(wy50080) mutant (d) at L4 stage. Arrows show PVD 2° branches without ER and arrowheads indicate PVD 2° branches with ER. Asterisks mark the PVD axon. Scale bars, 10 μm.e–hRepresentative ER morphology of PVD neuron in WT (e),atln-1(f), atln-1; ser-2Prom3::atln-1#2 (transgenic line #2) (g) andatln-1; ser-2Prom3::atln-1K80A#1(transgenic line #1) (h) at adult stage. Scale bars, 10 μm.i,jQuantification of ER 2° branches number. Values are mean and error bars are SEM,n= 46 for each genotype. *p< 0.05; ***p< 0.001 (two-sided student’sttest and Tukey’s multiple comparison test) 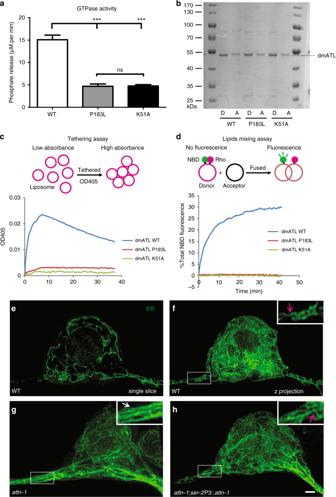Fig. 2 ATLN-1 regulates somatic ER network formation.aQuantification of GTPase activity of WT and mutant dmATLs. The activities were measured by phosphate release at saturating GTP concentrations of 0.5 mM. At least three repetitions were performed for each group. Values are mean and error bars are SEM. ns, not significant; ***p< 0.001 (Tukey’s multiple comparison test).bReconstitution ofDrosophilaWT, P183L, and K51A dmATL proteins into liposomes. Donor (D) and acceptor (A) vesicles with recombinant proteins were analyzed by SDS/PAGE and Coomassie blue staining. (c) Schematic illustration of liposome membrane tethering assay (upper panel). The clustering ofDrosophilaWT and mutant dmATL containing proteoliposomes (protein:lipid ratio 1:2,000) was measured by the light absorbance at a wavelength of 405 nm (lower panel).dSchematic illustration of lipid mixing assay (upper panel).DrosophilaWT and mutation dmATL were reconstituted at equal concentrations into donor and acceptor vesicles. GTP-dependent fusion of donor and acceptor vesicles was monitored by the dequenching of an NBD-labeled lipid in the donor vesicles (lower panel). Fusion was initiated by addition of GTP.eRepresentative 3D-SIM image of PVD somatic ER in a WT worm (single focal plane).f–hRepresentative 3D-SIM maximum-intensity-projection images of PVD somatic ER in WT (f),atln-1(g) andatln-1; ser-2P3::atln-1worms at adult stage. Insets show 2X magnified views. The magenta arrows indicate three-way junction and white arrows indicate parallel ER tubules. Scale bar, 1 μm 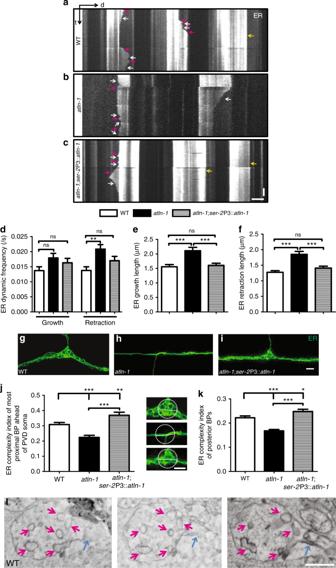Fig. 3 atln-1mutants show high level of ER retraction.a–cKymographs of ER (GFP::SP12) dynamic events in PVD 3° branches in WT (a),atln-1(b), andatln-1; ser-2P3::atln-1(c) worms at L4 stage. Magenta, white and yellow arrows indicate ER growth, retraction, and static events, respectively. Scale bar, 5 μm and 10 s.dQuantification of ER growth and retraction frequency. Values are mean and error bars are SEM. At least 200 events from more than 30 worms are quantified. ns, not significant, **p< 0.01 (Newman-Keuls multiple comparison test).e,fQuantification of ER growth (e) and retraction (f) length. Values are mean and error bars are SEM. At least 200 events from more than 30 worms are quantified. ns, not significant; ***p< 0.001 (Newman-Keuls multiple comparison test).g–iRepresentative 3D-SIM images of ER (GFP::SP12) complex structure at the most proximal branch point of the PVD anterior dendrite in WT (g),atln-1(h), andatln-1; ser-2P3::atln-1(i) worms.jQuantification of ER complexity index of the most proximal branching point. Values are mean and error bars are SEM,n> 40. **p< 0.01; ***p< 0.001 (Newman-Keuls multiple comparison test). To calculate the complexity index, we drew a circle of 1.6 μm diameter (dashed circle) at the branching point and a line within the circle along the dendrite trunk (dashed line). Complexity index = mean GFP intensity in the circle/mean GFP intensity on the line. Scale bars, 1 μm.kQuantification of ER complexity index at posterior branch points. Values are mean and error bars are SEM. At least 100 branch points from more than 30 worms are quantified. *p< 0.05; ***p< 0.001 (Newman-Keuls multiple comparison test).lScanning electron microscopy images from a serial EM pictures showing ER complex structure on a branch point in PVD of a WT worm. The magenta arrows indicate ER. The blue arrows indicate PVD 2° branches. Scale bar, 500 nm 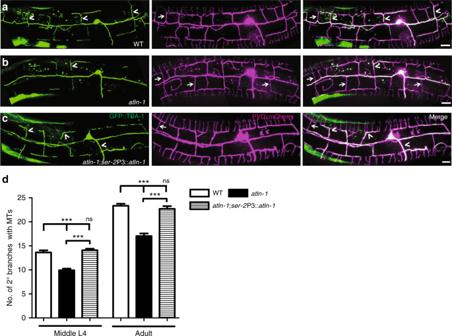Fig. 4 ATLN-1 affects the presence of MT in dendritic branches.a–cRepresentative confocal images of MTs (GFP::TBA-1) and dendritic morphology of PVD neuron (ser-2P3::mCherry) in WT (a),atln-1(b), andatln-1; ser-2Prom3::atln-1adult worms (c). Arrows show PVD 2° branches without MTs and arrowheads indicate PVD 2° branches with MTs. Scale bars, 10 μm.dQuantification of the number of 2° branches with MTs. Values are mean and error bars are SEM,n> 40. ns, not significant; ***p< 0.001 (Newman-Keuls multiple comparison test) All the strains and plasmids used are listed in Supplementary Table 1 , Supplementary Table 2 , Supplementary Table 3 , and Supplementary Table 4 . Fluorescent imaging, time-lapse imaging, Kymograph analysis For fluorescent imaging, worms were immobilized with 1 mg/ml levamisole in M9 buffer and transferred to a small glass slide or dish, then covered by a 3% (w/v) agar pad. Images were acquired using a 40X objective on a Zeiss Axio Observer Z1 microscope equipped with a 10X, 63X and 100X objective, an electron-multiplying charge-coupled device camera (Andor), a spinning-disk confocal scan head (Yokogawa CSU-X1 Spinning Disk Unit), and the 488- and 561 nm lines of a Sapphire CW CDRH USB Laser System. For ER dynamic analysis in Fig. 3 , 200 frames were taken for each movie at the speed of 1.54 frames per second. For MT dynamic analysis in Fig. 5 , 150 frames were taken for each movie at the speed of 1.19 frames per second. Movies were taken from PVD tertiary dendrites. For mitochondria fission analysis in Fig. 6 , 120 frames were taken for each movie at the speed of 0.2 frames per second. Movies were taken from the view in which PVD primary dendrite contained apparent long tubular mitochondria. 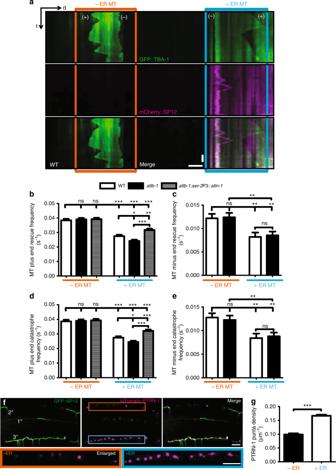Fig. 5 MT dynamics and numbers are affected by the ER.aKymographs recording the dynamic events of MT (GFP::TBA-1) and ER (mCherry::SP12) in 3° branches from a L4 stage WT animal. A blue box labels a +ER MT, while an orange box labels a –ER MT. MT’s plus end is marked by (+) and minus end is marked by (−). Scale bar, 5 μm and 15 s.b–eQuantification of dynamic parameters of MT plus ends (b,d) and minus ends (c,e). The frequency of rescue (b,c) and catastrophe (d,e) were plotted. Values are mean and error bars are SEM. At least 150 events from more than 30 worms are quantified. ns, not significant; *p< 0.05; **p< 0.01; ***p< 0.001 (Newman-Keuls multiple comparison test).fConfocal images showing tdTomato::PTRN-1 puncta in PVD 3° branches at adult stage. +ER (in blue box) means a 3° dendrite with ER present. -ER (in orange box) means the 3° branch without ER present. Scale bars, 10 μm.gQuantification of PTRN-1 puncta density in −ER and +ER 3° dendrites. Values are mean and error bars are SEM. At least 100 confocal views of PVD proximal regions from more than 40 worms are quantified. ***p< 0.001 (two-sided student’sttest) To measure the frequency of MT dynamic events, the term “catastrophe” is defined as the transition between polymerization and de-polymerization, whereas “rescue” describes the reverse transition. The frequency of dynamic events was calculated by counting the number of dynamic events dividing recording time. The growth and retraction length of ER was measured by the horizontal distance between adjacent transitions in kymographs. Movies and kymographs were generated and analyzed by ImageJ. Quantification and statistics For ER, dendritic and MT 2° branches quantification, worms at distinct stage were checked under 40X or 63X objectives using an Axio Imager M2 microscope (Carl Zeiss). For the quantification of 3-way junctions in PVD soma in Figs. 2 and 8 , a most recognizable region of 3 μm 2 (63 pixel × 31 pixel) at anterior primary dendrite initiation segment was selected, and this region would cover as more ER area as possible. Statistics analysis was performed using student’s t test, Tukey’s multiple comparison test, Newman-Keuls multiple comparison test or Chi-square test. Statistical analyses were generated and performed using Microsoft Excel and Prism 6 (GraphPad Software). 3D-SIM super-resolution microscopy and image analysis For 3D-SIM images, worms were immobilized with 3 mg/ml levamisole in M9 buffer and transferred to a small glass slide or dish, then covered by a 4–5% (w/v) agar pad. A half hour later, images were acquired on the DeltaVision OMX V3 imaging system (GE Healthcare) with a 100X/1.4NA oil objective (Olympus UPlanSApo), solid-state multimode lasers (488, 405, 561 nm) and electron-multiplying CCD (charge-coupled device) camera (Evolve 512 × 512, Photometrics). Serial Z-stack sectioning was done at 125 nm intervals for SIM mode. To obtain optimal images, immersion oils with refractive indices of 1.520 were used for PVD cell body or branch point on glass coverslips. The microscope is routinely calibrated with 100 nm fluorescent spheres to calculate both the lateral and axial limits of image resolution. SIM image stacks were reconstructed using softWoRx 6.1.1 (GE Healthcare) with the following settings: pixel 39.5 nm; channel-specific optical transfer function; Wiener filter constant 0.0010; discard Negative Intensities background; drift correction with respect to first angle; custom K0 guess angles for camera positions. The reconstructed images were further processed for maximum-intensity projections with softWoRx 6.1.1. Pixel registration was corrected to be less than 1 pixel for all channels using 100 nm Tetraspeck beads. GTPase activity assay Full-length, codon-optimized wild-type and mutant Drosophila ATL were expressed in in BL21 (DE3) cells as GST fusions. Expression was induced by the addition of 0.1 mM IPTG and continued for 24 h at 16 °C. Cells were lysed in A100 buffer [25 mM Hepes (pH 7.5), 100 mM KCl, 1 mM EDTA, 2 mM β-mercaptoethanol, and 10% (vol/vol) glycerol]. The membranes were pelleted by centrifugation and solubilized in Triton X-100. The GST fusion proteins were isolated with glutathione sepharose beads (GE Healthcare), washed, and eluted with 10 mM glutathione in A100 buffer with 0.1% Triton X-100. The GST tag was cleaved by Prescission protease (GE Healthcare) and was removed with glutathione agarose. GTPase assays were done with the Enzchek phosphate assay kit (Invitrogen). Reactions were performed in a 200 μL volume with 10 μL of 20× reaction buffer (1 M Tris·HCl/20 mM MgCl2, pH 7.5/2 mM sodium azide), 200 mM 2-amino-6-mercapto-7-methylpurine riboside, 1 unit/mL purine nucleoside phosphorylase (PNP), 2 μM ATL protein, or the indicated mutants, and incubated for 10 min at 37 °C in a 96-well plate (Nunc). Reactions were initiated by the addition of 0.5 mM GTP. The absorbance at 360 nm was measured every 31 s over 40 min at 37 °C by using a microplate reader (infinite M200 PRO). Rates of phosphate release were then calculated based on a standard curve. Liposomes tethering and lipids mixing assay Detergent-mediated reconstitution was used to integrate dmATL into preformed donor liposomes [82:15:1.5:1.5 mole percent of 1-palmitoyl-2-oleoyl-sn-glycero-3-phosphocholine (POPC):1, 2-dioleoyl-sn-glycero-3-phosphoserine (DOPS): NBD-1, 2-dipalmitoyl-sn-glycero-3-phosphoethanolamine (DPPE): rhodamine-DPPE] and acceptor liposomes (85:15 mole percent of POPC:DOPS). Lipids in chloroform were dried under a stream of N2 gas followed by further drying in a vacuum for 30 min. The lipid films were then re-suspended in A100 buffer to a final total lipid concentration of about 10 mM. Large unilamellar vesicles (LUVs) were formed by ten freeze-thaw cycles in liquid N2 and room temperature water. Uniform-sized LUVs were formed by extrusion through polycarbonate filters with 100-nm pore size (Avanti Polar Lipids). Wild-type and mutant Drosophila ATL proteins were mixed with preformed liposomes at an effective detergent to lipid ratio of ~1:1. Proteins and lipids were allowed to mix for 1 h at 4 °C. 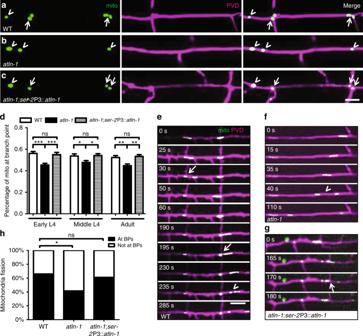Fig. 6 ATLN-1 modulates mitochondria dynamics in dendrites.a–cMitochondria distribution in PVD primary dendrites in WT (a),atln-1(b) andatln-1; ser-2Prom3::atln-1(c) worms at adult stage. Arrows indicate mitochondria at branch points. Arrowheads indicate mitochondria which are not localized at branch points. Scale bar, 5 μm.dQuantification of the percentage of mitochondria localized at branch points. Values are mean and error bars are SEM,n> 25 for each genotype. ns, not significant; *p< 0.05; **p< 0.01; ***p< 0.001 (Newman-Keuls multiple comparison test).e–gTime-lapse images of mitochondria fission in WT (e),atln-1(f), andatln-1; ser-2P3::atln-1(g) worms. The arrows indicate mitochondria fission events at branch points. The arrowheads indicate mitochondria fission events outside of branch points. Scale bar, 10 μm.hQuantification of mitochondria fission events at and outside of branch points.n= 40–50. ns, not significant; *p< 0.05 (Chi-square test) Detergent was removed by adding BioBeads SM-2 adsorbant beads (BioRad) five times every hour, and incubating overnight after the final addition of beads. 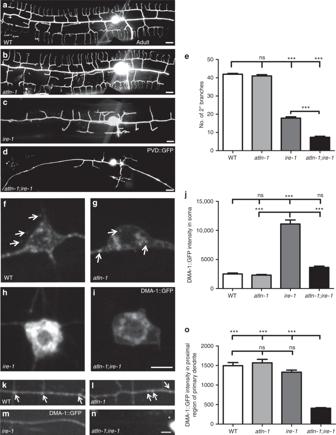Fig. 7 atln-1functions synergistically withire-1.a–dRepresentative confocal images of PVD (ser-2P3::GFP) morphology in WT (a),atln-1(b),ire-1(ok799) (c) andatln-1; ire-1(d) worms at adult stage. Scale bars, 10 μm.eQuantification of the number of PVD 2° branches. Values are mean and error bars are SEM,n> 40. ns, not significant; ***p< 0.001 (Newman-Keuls multiple comparison test).f–iConfocal images of DMA-1::GFP in PVD cell body in WT (f),atln-1(g),ire-1(h), andatln-1; ire-1(i) worms. Arrows indicate DMA-1::GFP puncta. Scale bar, 5 μm.jQuantification of DMA-1::GFP fluorescence intensity in PVD cell body. Values are mean and error bars are SEM,n= 40–50. ns, not significant; ***p< 0.001 (Newman-Keuls multiple comparison test).k–nConfocal images of DMA-1::GFP in anterior primary dendrite around the PVD soma in WT (k),atln-1(l),ire-1(m), andatln-1; ire-1(n) worms. Arrows indicate DMA-1::GFP puncta. Asterisk marks cell body. Scale bar, 5 μm.oQuantification of DMA-1::GFP fluorescence intensity of primary dendrites in (k–n). Values are mean and error bars are SEM,n= 40–50. ns, not significant; ***p< 0.001 (Tukey’s multiple comparison test) 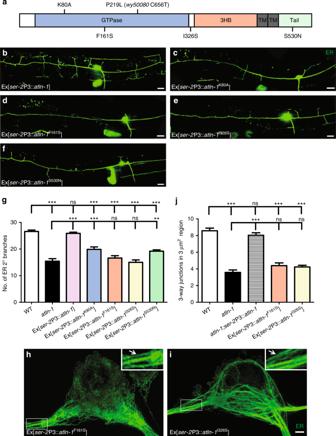Fig. 8 HSP disease alleles of Atlastin-1 affect ER morphology.aSchematic diagram of ATLN-1 protein domains. K80A,wy50080(P219L) and HSP related disease mutations are showed.b–fRepresentative ER morphology in Ex[ser-2P3::atln-1] (b), Ex[ser-2P3::atln-1K80A] (c), Ex[ser-2P3::atln-1F161S] (d), Ex[ser-2P3::atln-1I326S] (e) and Ex[ser-2P3::atln-1S530N] (f) transgenic adult worms. Scale bars, 10 μm.gQuantification of ER 2° branches number. Values are mean and error bars are SEM,n= 40–50. ns, not significant; **p< 0.01; ***p< 0.001 (Tukey’s multiple comparison test).h,iRepresentative maximum-intensity-projection 3D-SIM images of ER in PVD soma in Ex[ser-2P3::atln-1F161S] (g) and Ex [ser-2P3::atln-1I326S] (h) transgenic adult worms. Insets show 2X magnified views. Scale bar, 1 μm.jQuantification of 3-way junctions in a 3 μm2region at anterior primary dendrite initiation segment (the dashed boxes inhandi). Values are mean and error bars are SEM,n> 30. ns, not significant; ***p<0.001 (Newman-Keuls multiple comparison test) Insoluble protein aggregates were pelleted by centrifugation of the samples in an Eppendorf microcentrifuge. For Liposomes tethering assay, GTP was added at 1 mM concentration to proteoliposomes containing WT and mutant ATL. Absorbance at 405 nm was measured on an infinite M200 PRO Microplate Reader. The absorbance before nucleotide addition was set to zero. For lipids mixing assay, donor and acceptor vesicles were mixed at a 1:3 ratio in A100 supplemented with 5 mM MgCl 2 . GTP was added to 1 mM to start the fusion reaction, and the fluorescence intensity of NBD was monitored with an excitation of 460 nm and emission of 538 nm using a SpectraMax M5 Microplate Reader or Biotek Synergy 4 plate reader. The maximal NBD fluorescence was determined after addition of dodecyl maltoside. The initial NBD fluorescence prior to nucleotide addition was set to zero, and the initial background fluorescence was subtracted from the raw fluorescence readings, and these values are expressed as percentages of the maximum fluorescence after detergent addition. Reporting summary Further information on experimental design is available in the Nature Research Reporting Summary linked to this article.